Chemical structures of hydrazine-treated graphene oxide and generation of aromatic nitrogen doping Chemically modified graphene platelets, produced via graphene oxide, show great promise in a variety of applications due to their electrical, thermal, barrier and mechanical properties. Understanding the chemical structures of chemically modified graphene platelets will aid in the understanding of their physical properties and facilitate development of chemically modified graphene platelet chemistry. Here we use 13 C and 15 N solid-state nuclear magnetic resonance spectroscopy and X-ray photoelectron spectroscopy to study the chemical structure of 15 N-labelled hydrazine-treated 13 C-labelled graphite oxide and unlabelled hydrazine-treated graphene oxide, respectively. These experiments suggest that hydrazine treatment of graphene oxide causes insertion of an aromatic N 2 moiety in a five-membered ring at the platelet edges and also restores graphitic networks on the basal planes. Furthermore, density-functional theory calculations support the formation of such N 2 structures at the edges and help to elucidate the influence of the aromatic N 2 moieties on the electronic structure of chemically modified graphene platelets. In the 1960s, hydrazine (NH 2 NH 2 ) was used to chemically reduce thin graphite oxide (GO) particles [1] , [2] ; Ruoff and co-workers [3] developed the use of hydrazine to reduce individual graphene oxide platelets four decades later. For the last half decade, among several chemical reductants [4] , [5] , hydrazine has been the most commonly used reductant due to its ease of use (for example, via a one-pot synthesis in either liquid or gas phase) and its ability to achieve a high degree of reduction of graphene oxide without the need for further treatment [3] , [6] , [7] , [8] . Hydrazine-treated graphene oxide (chemically reduced graphene oxide, 'CReGO') [3] is one of the most promising graphene-based materials for several applications, such as polymer composites, ultracapacitors, rechargeable batteries, chemical/biosensors and thin films [9] , [10] , [11] , [12] , [13] , [14] . A large fraction of the oxygen-based functional groups of graphene oxide are removed by exposure to hydrazine; however, the resulting graphene materials contain a small amount of O and N atoms (with approximate C/O and C/N ratios of 10 and 22, respectively) [3] , [6] . The presence of these heteroatoms on the 'graphene' platelets—namely, electron donating N atoms and electron withdrawing O atoms—may create a doping effect that considerably affects their electronic structure [15] . Also, chemical moieties containing heteroatoms or heterocycles can be utilized to open a new path to selective chemical modifications of graphene-based systems. However, despite the use of CReGO in a variety of different ways [9] , [10] , [11] , the chemical identities of the functional groups containing those heteroatoms have not yet been fully determined. 13 C solid-state nuclear magnetic resonance (SSNMR) spectroscopy may be the most powerful method to study the detailed chemical structures of graphene-based materials such as graphene oxide, GO, reduced graphene oxide and other chemically modified graphenes (CMGs) [16] , [17] . However, the low natural abundance (1.1%) of the 13 C isotope results in a low signal-to-noise ratio, which, along with the broad peaks typically observed from CMGs, precludes the use of multidimensional SSNMR. This was the motivation for our recent work, which used 99% 13 C-labelled graphite made by chemical vapour deposition (CVD) as the precursor to 13 C-labelled GO, which was studied using 13 C SSNMR [18] , [19] . This investigation revealed that hydroxyl, 1,2-epoxide and sp 2 carbons on the basal planes [20] are directly bonded to each other in GO. It has been proposed that sp 2 networks in GO are terminated with carboxyl and ketone groups, predominately at the edges of the structure [21] . Separately, the existence of five- or six-membered lactol rings at the edges of GO has been suggested by Gao et al [22] . While considerable structural information has been obtained for GO, few structural details, especially at the platelet edges, have been obtained for CReGO or unexfoliated GO reduced by hydrazine, the latter of which we define as reduced graphite oxide or 'RGO'. For SSNMR measurements, a protocol to produce 13 C- and 15 N-labelled RGO by reducing 13 C-labelled GO with 15 N-hydrazine monohydrate was developed, and 1 H/ 13 C/ 15 N triple-resonance SSNMR experiments were performed on the samples. SSNMR spectroscopy of N typically requires the use of isotopically labelled samples because of the low natural abundance of 15 N (~0.4%) and also large quadrupolar interactions of naturally abundant 14 N nuclei. Herein, we present new structural insight into reduced graphene oxide materials, revealed by 13 C- and 15 N rotational-echo double-resonance (REDOR) SSNMR experiments [23] , [24] on 13 C- and 15 N-labelled RGO as well as by X-ray photoelectron spectroscopy (XPS) measurements on unlabelled, hydrazine-treated graphene oxide. This work helps to provide a deeper understanding of the chemical structures and electronic properties of reduced graphene oxides. NMR study of isotope-labelled RGO samples A 13 C-labelled graphite film was grown by CVD of 13 C-enriched methane on Ni foil as described previously [18] . Raman spectroscopy confirmed that the as-grown graphite film was of high quality and highly enriched (99%) in the 13 C isotope ( Supplementary Fig. S1 ) [18] . As expected, the first-order G-band was observed at 1,518 cm −1 , while the D-band typically detected at 1,297 cm −1 was completely absent. This result indicates high-quality films and an enrichment of approximately 99% 13 C. 13 C-labelled graphite film was removed from the Ni substrate by scotch tape, then rinsed and sonicated in acetone. As shown in Supplementary Figure S1 , the graphite film was cut into small pieces (10–50 μm). This 13 C-labelled graphite was then oxidized to 13 C-labelled GO, and subsequently reduced using 98% 15 N-labelled hydrazine monohydrate to produce 13 C-, 15 N-labelled RGO (see the Methods section for experimental details). 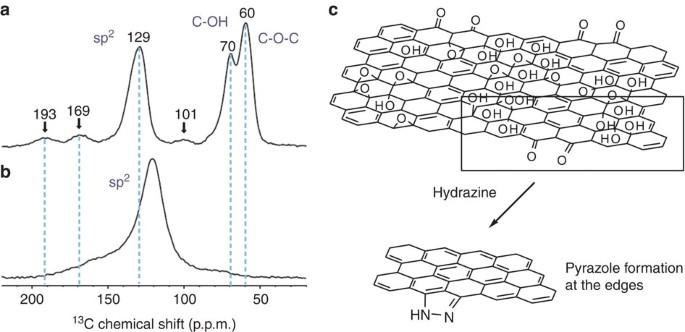Figure 1: Chemical structures of labelled samples before and after hydrazine treatment. 13C MAS SSNMR spectra of (a)13C-labelled GO and (b)13C- and15N-labelled RGO. The spectrum inawas reproduced fromFigure 1ain our previous work by Caiet al.18Reprinted with permission from AAAS. All the spectra were obtained with direct13C excitation by a π/2 pulse at a13C NMR frequency of 100.643 MHz and with 20 kHz MAS. (c) A schematic illustrating pyrazole formation at the edges of the platelets during hydrazine treatment of graphene oxide (–COOH groups at the platelet edges have been omitted for clarity). Figure 1 shows high-resolution magic angle spinning (MAS) 13 C-SSNMR spectra of (a) the labelled GO and (b) the labelled RGO samples. High-resolution SSNMR spectroscopy using MAS has been used to study the chemical structures of GO [3] , [18] , [22] . A spectrum of the labelled RGO sample ( Fig. 1b ) shows an excellent signal-to-noise ratio, despite the small sample quantities of approximately 2 mg and a relatively short acquisition time of 21 min. Notably, obtaining a spectrum of similar quality from an unlabelled sample would require signal accumulation for nearly 140 days. There are several obvious spectral changes from the samples before and after hydrazine treatment. In Figure 1a , there is a weaker peak at 193 p.p.m., which was previously assigned to ketone groups (RR'C=O) at the edges of the platelets [22] . The edge structures could be present around hole defects or torn edges in the interior of the platelets [25] , [26] . The high sensitivity resulting from our novel isotope labelling method is especially useful for SSNMR analysis of important species with lower populations. Interestingly, the peak at 193 p.p.m. disappeared in Figure 1b , suggesting that the changes occurred in the chemical structure at the edges. As GO is thermally unstable, thermal treatment of GO under our reaction conditions might lead to changes in the chemical structure of GO. However, stirring GO in water at 80 °C without hydrazine resulted in little change of the chemical structure of GO, as shown in Supplementary Figure S2 . These results confirm that hydrazine is responsible for the changes in the chemical structure of graphene oxide. Figure 1: Chemical structures of labelled samples before and after hydrazine treatment. 13 C MAS SSNMR spectra of ( a ) 13 C-labelled GO and ( b ) 13 C- and 15 N-labelled RGO. The spectrum in a was reproduced from Figure 1a in our previous work by Cai et al . [18] Reprinted with permission from AAAS. All the spectra were obtained with direct 13 C excitation by a π/2 pulse at a 13 C NMR frequency of 100.643 MHz and with 20 kHz MAS. ( c ) A schematic illustrating pyrazole formation at the edges of the platelets during hydrazine treatment of graphene oxide (–COOH groups at the platelet edges have been omitted for clarity). Full size image Advanced SSNMR experiments correlating the connectivity of 13 C and 15 N have been used for 13 C- and 15 N-labelled biomolecules [27] , [28] , [29] ; however, for graphene-based materials, such SSNMR experiments have not been performed to date, partly because of the difficulties in the preparation of appropriate samples. 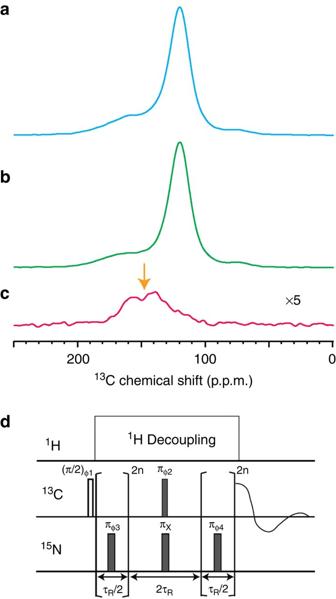Figure 2:13C REDOR SSNMR measurement of labelled RGO. 13C MAS SSNMR spectra with a π/2-pulse excitation of13C- and15N-labelled RGO, (a) without and (b) with dipolar dephasing by13C–15N REDOR during a period of 1.6 ms. (c) The difference spectrum ofaandb. Note that the vertical scale incis magnified five times, compared with that ofaandb. The spectra inaandbwere collected with the pulse sequence shown (d), (a) without and (b) with15N π-pulse trains. Although the13C signal intensities for both control and dephased spectra are mildly modulated by13CT2relaxation and13C–13C J-coupling, the difference spectrum inchighlights a spectrum of13C species within a few bonds from15N atoms. The phase cycles indare as follows: φ1=x, −x, y, −y; φ2=y, y, −x, −x. The receiver phase was cycled as x, −x, y, −y. The phases for φ3and φ4in the rotor-synchronous π-pulse trains were incremented after every π-pulse, following the XY-16 phase cycle (x, y, x, y, y, x, y, x, −x, −y, −x, −y, −y, −x, −y, −x). τRdenotes one rotation period of magic angle spinning. In this work, we acquired the 13 C MAS SSNMR spectra without and with 13 C– 15 N dipolar dephasing using a REDOR pulse sequence, as shown in Figure 2a,b , respectively. Details on the pulse sequence are provided in Figure 2d (refs 23 , 24 ). The 13 C atoms associated with 15 N atoms lose their signal in the 13 C MAS spectrum with 13 C– 15 N dephasing. Subtraction of Figure 2b from Figure 2a shows NMR signals of the 13 C atoms that are one or at most two bonds away from 15 N atoms [24] . The resulting difference spectrum, shown in Figure 2c , reveals a new spectral feature around 150 p.p.m. (labelled with an arrow in Fig. 2c ), which has not been reported previously. The broad signal with two maxima at 140 and 157 p.p.m. cannot be observed as a separate peak in the spectrum shown in Figure 2a without 13 C– 15 N dephasing, as they are overlapped with a major peak centred at 118 p.p.m. In an attempt to eliminate the effect of any associated 15 N-labelled contaminants resulting from the 15 N-labelled hydrazine treatment, the RGO sample was thoroughly washed with acetone and subsequently dried under high vacuum; then the REDOR experiment was repeated. The REDOR experiment on the washed RGO sample yielded an almost identical result to that shown in Figure 2 (data not shown). Because the natural abundance of 15 N is extremely low, this observation suggests that the RGO contains 15 N species that originate from 15 N-labelled hydrazine and that the 15 N species are likely to be chemically bonded to 13 C species of RGO. We found this peak at approximately 150 p.p.m. for another labelled sample, which was prepared from a separate batch ( Supplementary Fig. S3 ). Figure 2: 13 C REDOR SSNMR measurement of labelled RGO. 13 C MAS SSNMR spectra with a π/2-pulse excitation of 13 C- and 15 N-labelled RGO, ( a ) without and ( b ) with dipolar dephasing by 13 C– 15 N REDOR during a period of 1.6 ms. ( c ) The difference spectrum of a and b . Note that the vertical scale in c is magnified five times, compared with that of a and b . The spectra in a and b were collected with the pulse sequence shown ( d ), ( a ) without and ( b ) with 15 N π-pulse trains. Although the 13 C signal intensities for both control and dephased spectra are mildly modulated by 13 C T 2 relaxation and 13 C– 13 C J-coupling, the difference spectrum in c highlights a spectrum of 13 C species within a few bonds from 15 N atoms. The phase cycles in d are as follows: φ 1 =x, −x, y, −y; φ 2 =y, y, −x, −x. The receiver phase was cycled as x, −x, y, −y. The phases for φ 3 and φ 4 in the rotor-synchronous π-pulse trains were incremented after every π-pulse, following the XY-16 phase cycle (x, y, x, y, y, x, y, x, −x, −y, −x, −y, −y, −x, −y, −x). τ R denotes one rotation period of magic angle spinning. Full size image Given these observations, we suggest that the 13 C NMR peak around 150 p.p.m. can be attributed to pyrazole groups—aromatic five-membered rings with two adjacent N atoms as shown in Figure 1c —which usually show 13 C NMR signals between 150 and 160 p.p.m. [30] Pyrazole groups have been produced by the reaction of diketone groups with primary amine moieties [31] . In addition, the formation of pyrazole groups from the reaction between hydrazine (one of the primary amine moieties) and diketone groups has been well established; for example, see the reaction shown in Supplementary Figure S4 (ref. 31 ). Alternatively, the new 13 C NMR peaks around 150 p.p.m. may be also assigned to C=N bonds. Hydrazone groups, which contain non-aromatic C=N double bonds, have been produced by the reaction between hydrazines and ketones or aldehydes as shown in Supplementary Figure S4 (refs 32 , 33 ). In either case, the reactions may take place at the ketone groups of GO via nucleophilic attack by the hydrazine molecules. Consequently, both reactions can explain the complete removal of the ketone peak in the 13 C NMR spectrum. However, it is difficult to distinguish between pyrazole and hydrazone groups based on the chemical shifts in the 13 C NMR spectrum. 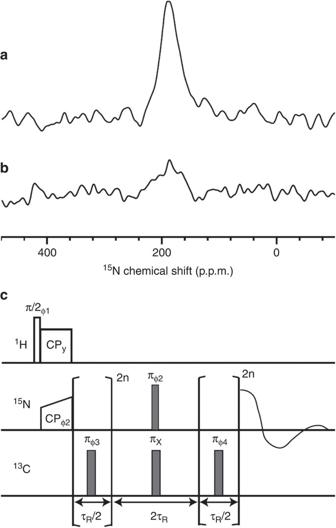Figure 3:15N REDOR SSNMR measurement of labelled RGO. 15N CPMAS SSNMR spectra of13C- and15N-labelled RGO (a) without and (b) with13C–15N dipolar dephasing by (c) a REDOR pulse sequence with a dephasing period of 1.6 ms, (a) without and (b) with15N π-pulse trains for the15N channel. Although the15N-signal intensities for both control and dephased spectra are mildly modulated by15NT2relaxation, residual1H–15N dipolar couplings under fast MAS, and15N–15N J-coupling, the signal of15N species within a few bonds from13C are substantially suppressed by15N–13C dipolar couplings when a13C π-pulse train is applied as shown inb. The phase cycles incare as follows: φ1=x, −x; φ2=y, y, −x, −x. The receiver phase was cycled as x, −x, y, −y. The phases for φ3and φ4in the rotor-synchronous π-pulse trains were incremented after every π-pulse, following the XY-16 phase cycle. τRdenotes one rotation period during magic angle spinning. The 15 N MAS SSNMR spectrum of the 13 C- and 15 N-labelled material was obtained with cross-polarization (CP) from 1 H spins and is shown in Figure 3a . To the best of our knowledge, this is the first report of a 15 N NMR study on a graphene-based material. The spectrum in Figure 3a shows a broad peak centred at approximately 190 p.p.m., which can be assigned to pyrazole moieties [34] . Because of the short contact time of 0.35 ms used in the CP period, the signal is likely due to protonated 15 N atoms. From the data, an N atom (–NH2 moiety) in a hydrazone group (–C=N–NH 2 ) can be ruled out because NMR signals corresponding to –NH 2 groups are usually observed between 0 and 100 p.p.m. in 15 N NMR (ref. 30 ). Figure 3b shows the 15 N MAS spectrum with 13 C– 15 N dipolar dephasing, acquired using a REDOR pulse sequence ( Fig. 3c ). It can be seen that the peak at 190 p.p.m. is considerably decreased by 13 C– 15 N dephasing, suggesting covalent attachment of the 15 N species on 13 C atoms. On the basis of the SSNMR experiments with labelled RGO samples, we believe this suggests the formation of aromatic pyrazole groups at the edges of platelets after hydrazine treatment. Although the defect structures in the interior of the platelets are not well understood, these pyrazole rings could be generated at the edges around the interior defects. Figure 3: 15 N REDOR SSNMR measurement of labelled RGO. 15 N CPMAS SSNMR spectra of 13 C- and 15 N-labelled RGO ( a ) without and ( b ) with 13 C– 15 N dipolar dephasing by ( c ) a REDOR pulse sequence with a dephasing period of 1.6 ms, ( a ) without and ( b ) with 15 N π-pulse trains for the 15 N channel. Although the 15 N-signal intensities for both control and dephased spectra are mildly modulated by 15 N T 2 relaxation, residual 1 H– 15 N dipolar couplings under fast MAS, and 15 N– 15 N J-coupling, the signal of 15 N species within a few bonds from 13 C are substantially suppressed by 15 N– 13 C dipolar couplings when a 13 C π-pulse train is applied as shown in b . The phase cycles in c are as follows: φ 1 =x, −x; φ 2 =y, y, −x, −x. The receiver phase was cycled as x, −x, y, −y. The phases for φ 3 and φ 4 in the rotor-synchronous π-pulse trains were incremented after every π-pulse, following the XY-16 phase cycle. τ R denotes one rotation period during magic angle spinning. Full size image XPS measurements and calculations on XPS spectra As the SSNMR spectra of the unlabelled hydrazine-treated graphene oxide showed a limited signal-to-noise ratio and broad signals, XPS was measured on two groups of unlabelled hydrazine-treated graphene oxide samples: graphene oxide platelets in homogeneous colloidal suspensions that were treated with hydrazine and then vacuum filtered to create free-standing 'paper-like' materials [35] , [36] , and a film composed of graphene oxide platelets spin-coated on glass and then treated with hydrazine vapour. 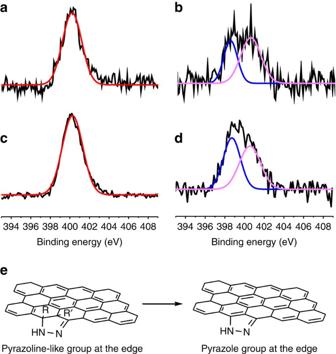Figure 4: Chemical structures of unlabelled samples before and after hydrazine treatment. N1snarrow scans in XPS spectra of reduced graphene oxide samples; ina, the reduced graphene oxide is a paper-like material produced by filtration of a suspension of hydrazine-treated graphene oxide platelets; (b), sample (a) following a thermal annealing treatment; (c), a hydrazine vapour-treated graphene oxide film; and (d), sample (c) following a thermal annealing treatment. (e) A schematic diagram for pyrazoline-to-pyrazole conversion at the edges. In both cases we observed similar N 1s spectra indicating pyrazole moieties, as shown in Figure 4 . Figure 4: Chemical structures of unlabelled samples before and after hydrazine treatment. N 1s narrow scans in XPS spectra of reduced graphene oxide samples; in a , the reduced graphene oxide is a paper-like material produced by filtration of a suspension of hydrazine-treated graphene oxide platelets; ( b ), sample ( a ) following a thermal annealing treatment; ( c ), a hydrazine vapour-treated graphene oxide film; and ( d ), sample ( c ) following a thermal annealing treatment. ( e ) A schematic diagram for pyrazoline-to-pyrazole conversion at the edges. Full size image The N 1s spectra of the 'as-prepared' samples in Figure 4a,c show one symmetrical peak around 400 eV, which can be assigned to pyrazoline groups (non-aromatic five-membered rings) rather than pyrazole groups, as discussed below. Although the two N atoms in pyrazoline groups are not identical, the two N 1s peaks in XPS appear at almost the same position, resulting in the generation of one overlapped peak [37] . As shown in Figure 4b,d , thermal annealing (as described in the Methods section) splits the N 1s peak into two well-resolved lines at 398.6 and 400.5 eV, suggesting that two N atoms have considerably different chemical environments as observed in pyrazole groups. While the twofold-coordinated N atom in the pyrazole group has a localized lone pair of electrons, the threefold-coordinated N associates with delocalized electrons in the aromatic ring. Density-functional theory (DFT) calculations [37] were performed on pyrazole groups at the edges of graphene platelets for understanding their chemical structure, particularly associated with the experimental XPS peak separation of 1.9 eV (ref. 38 ). The N–N moiety of the pyrazole ring in a graphene nanoribbons with zigzag edges (zGNR) consists of two different N atoms; one is twofold coordinated with a lone pair of electrons, and the other is threefold coordinated with one hydrogen atom in the sp 2 planar configuration, as shown in Supplementary Figure S5 . The former is pyridinic-like and the latter is quaternary-like. The two N atoms should be in different ionization states with different N 1s core-level binding energies as in the pyrazole molecule. Our first-principles DFT calculations give a core-level separation of 1.52 eV for pyrazolated zGNR, consistent with the experimental XPS peak separation of 1.9 eV. These values are also very close to 1.59 and 1.8 eV for pyrazole molecules obtained from DFT calculation and XPS measurements, respectively. Unlike the zGNR model, GO may not be perfectly flat because there is often a considerable amount of residual oxygen after a typical hydrazine treatment. If this is indeed the case, the tertiary N should undergo out-of-plane relaxation as in an amine group with a lone pair, as shown in Supplementary Figure S5 . Then, the core level of the amine-like N should nearly coincide with that of the pyridinic-like N, at around 400 eV. Our calculations for a zGNR distorted by two extra hydroxyls results in nearly coincident core levels. The core-level separation is only 0.22 eV, which can be viewed as a single peak in the XPS measurement. The theoretical core-level separation for pyrazoline molecules is 0.17 eV. Therefore, we can explain the single-to-double transition of N 1s XPS peaks on thermal treatment as follows. The hydrazine treatment of GO would incorporate many N–N moieties into the RGO sample. Because of incomplete reduction of RGO, the incorporated N–N moieties have an sp 3 configuration as in pyrazoline groups. After further reduction of RGO by thermal treatment, the N–N moieties in RGO are more akin to sp 2 pyrazole groups. Calculation on reaction pathways and electronic structures To understand the formation mechanism of the pyrazole groups, we considered several possible reaction routes using graphene nano-ribbons with zGNR as shown in equations (1,2,3 and 4). DFT calculations also support the formation of five-membered rings at the edges after hydrazine treatment. Two zigzag edge sites are functionalized as represented by dashes inside the parentheses. ΔE is the reaction energy from the DFT calculations, with a negative reaction energy indicating an exothermic reaction. When a diketone is presented on the zigzag edge, the formation of a pyrazole group is very likely as the reaction energy is about −2 eV, as shown in equation (1). Other types of edge structures containing ketone or hydroxyl groups can also be converted into pyrazole rings and show non-negligible exothermic reaction energies, as shown in equations (2) and (3). On the contrary, the formation of a hydrazone group is not energetically favourable with an endothermic reaction energy of 0.38 eV, as shown in equation (4). This is consistent with our experimental observations. It is possible that hydrazine-assisted chemical reduction produced N atom-free species at the edges, which, in part, might contribute to the disappearance of the NMR peak at 190 p.p.m. that was previously assigned to C=O groups at the platelet edges. However, this mechanism is not sufficient to explain the presence of pyrazole/pyrazoline groups as suggested by our SSNMR and XPS data. In the field of graphene-based materials, the term 'reduction' typically refers to the removal of oxygen atoms from graphene oxide/GO. However, pyrazole formation at the edges is more properly referred to as a 'substitution' rather than a 'reduction' ( Fig. 1c ). The aromaticity of the pyrazole moiety should enhance electron conduction because of the reduced band gap and the delocalized electronic states associated with the N in the sp 2 configuration. 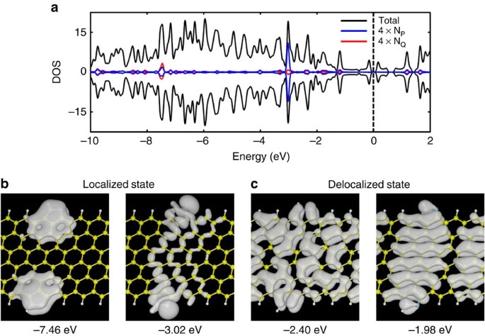Figure 5: Theoretical calculation on electronic structures of RGO materials with N2doping at the edges. (a) Density of states (DOS) of a zigzag graphene nanoribbon with pyrazoles at both the edges, and (b,c) a set of charge density plots of N2-related electronic states at several energies for (b) localized states and (c) delocalized states. Figure 5 illustrates the total and local densities of states of zGNR with pyrazole groups at the edges, and several electronic states that are associated with the N 2 pyrazole moieties. We can clearly identify the localized lone pair electronic state at −3 eV (below the Fermi level), which corresponds to the pyridinic N (N P ). The electronic state of the sp 2 or quaternary N (N Q ) can be found at several energies, for example, −7.5, −2.4 and −2.0 eV. The state at −7.5 eV is pentagonal, as in the aromatic pyrazole. The N Q electronic states near the Fermi level are well hybridized with the graphene bulk states. Consequently, aromatic N 2 doping (particularly, N Q ) strongly influences the electronic structures of hydrazine-treated graphene oxide materials. Figure 5: Theoretical calculation on electronic structures of RGO materials with N 2 doping at the edges. ( a ) Density of states (DOS) of a zigzag graphene nanoribbon with pyrazoles at both the edges, and ( b , c ) a set of charge density plots of N 2 -related electronic states at several energies for ( b ) localized states and ( c ) delocalized states. Full size image The SSNMR measurements revealed the presence of other chemical groups on the labelled RGO sample. A peak corresponding to sp 2 -bound 13 C atoms in GO at roughly 130 p.p.m. had shifted upfield to 118 p.p.m. as shown in Figure 1b . This is consistent with previous reports on the SSNMR spectra of unlabelled, reduced graphene oxides [3] , [22] . The peak shift indicates a greater amount of sp 2 conjugation in RGO than in GO, thus suggesting that the sp 2 network was restored by hydrazine treatment. A peak at approximately 70 p.p.m. corresponding to hydroxyl (–COH) groups [18] , [19] was nearly removed, while a peak at 60 p.p.m., previously assigned to 1,2-epoxide functionalities [18] , [19] , was completely suppressed after hydrazine treatment. This suggests that hydroxyl groups on the basal plane were mostly removed and 1,2-epoxide groups on the basal planes were completely removed by the hydrazine treatment (within the detection limit of these NMR measurements). In other words, the basal planes of GO have largely been reduced by the hydrazine treatment. Although the mechanism is not well understood, the reduction of GO is generally believed to restore the sp 2 networks on the basal planes while reducing the concentration of hydroxyl and 1,2-epoxide groups. The region around 170 p.p.m. in Figure 1b , which was previously assigned to carboxyl groups (–COOH) at the edges of platelets of RGO [18] , [19] , overlaps with a tail of the peak at 150 p.p.m. Consequently, it is difficult to conclusively determine whether carboxyl groups remain in the RGO sample based on the peak assigned to them. It is well known that carboxyl groups can be reduced to hydroxyl groups by reaction with strong reductants such as lithium aluminium hydride [32] , [33] . However, in the case of hydrazine treatment under the reaction conditions used here, the reduction of carboxyl groups to hydroxyl groups could be ruled out due to the absence of a peak corresponding to hydroxyl groups in the 13 C NMR spectrum of labelled RGO. In addition, it may be expected that the carboxyl groups can be converted to amide groups (–CO–NH–NH 2 ) by reaction with hydrazine. However, the 15 N SSNMR spectra did not indicate the presence of –NH 2 groups, thus suggesting that no amide groups were generated. In conclusion, we investigated the chemical structures of hydrazine-treated graphene oxide/GO, which is one of the most widely used graphene-based materials, using SSNMR spectroscopy and XPS. We first produced 13 C- and 15 N-labelled RGO materials by reaction of 13 C-labelled GO with 15 N-labelled hydrazine monohydrate. The isotope-labelled materials showed tremendously improved SSNMR signals relative to unlabelled material and we found that the hydrazine treatment caused the formation of pyrazole groups—aromatic five-membered rings with two adjacent N atoms—at the edges of resulting platelets. Furthermore, XPS experiments on unlabelled, hydrazine-treated graphene oxide revealed the formation of five-membered pyrazoline or pyrazole rings (after heat treatment) at the edges. The evidence of chemical substitution by hydrazine may offer a novel path to selective chemical modifications at the edges of graphene platelets for graphene-based systems. For example, an acidic proton in the pyrazole rings could be activated by treatment with a strong base for further modification [31] . The methods and results presented here show that isotopic labelling with NMR-active nuclei such as 13 C and 15 N, particularly when combined with other spectroscopic methods such as XPS, can provide detailed insight into the chemical structure of CMGs. The SSNMR spectra of 13 C- and 15 N-labelled RGO also showed almost complete removal of epoxy and hydroxyl groups, and significant restoration of the sp 2 network on the basal planes. On the basis of our analysis, we suggested that the term 'hydrazine-reduced/substituted graphene oxide' is more correct and descriptive than 'hydrazine-reduced graphene oxide' which, to date, has generally been used in the peer-reviewed literature to refer to this material. Preparation of 13 C-labelled graphite Uniformly 13 C-labelled graphite films were prepared using a cold-wall CVD system, as described previously [18] . The graphite was obtained by precipitation from the Ni foil during cooling, and formed on both sides of the Ni foil. The 13 C-labelled graphite film was removed from the Ni substrate using scotch tape. The graphite films on the scotch tape were immersed in acetone for 1 day to dissolve the tape, then sonicated for 30 min. The supernatant was decanted and this dissolving and decanting process was repeated two more times. After filtration followed by washing with dimethylformamide, ethanol and acetone, three times each, the product was dried in the oven (60 °C) for 2 days, and 13 C-labelled graphite flake was obtained. Preparation of 13 C- and 15 N-labelled RGO 13 C-labelled GO was produced by the modified Hummers method [39] . Control experiments were used to determine the proper amounts of hydrazine monohydrate to add for the creation of RGO samples. We tested the effect of the amount of hydrazine monohydrate relative to GO in liquid-phase reaction without isotope labelling. It was found that 1 μl of hydrazine monohydrate is sufficient to reduce 3 mg of GO (data not shown). Consequently, we used the same ratio of hydrazine monohydrate to GO with the labelled chemicals in this work. The 13 C-labelled graphite (60 mg) was added to a flask filled with H 2 SO 4 (30 ml), then the mixture was sonicated for 2 h. Solid KMnO 4 (300 mg, 99.2%, Fisher Scientific) was then slowly added to the flask in an ice bath. After addition of the KMnO 4 , the flask was immersed in a water bath at 35 °C, and stirred with a magnetic bar for 24 h. Deionized water (150 ml) was added to the flask in the ice bath, followed by stirring in this ice bath for 1 h. The flask was then taken off the ice bath and stirred at room temperature for 2 h. Hydrogen peroxide (30 wt% in water, Sigma-Aldrich) was then added to the mixture until no further gas evolution was observed, followed by stirring for 2 h. The mixture was then filtered using an Anodisc membrane filter (47 mm in diameter, 0.2-μm pore size, Whatman, Middlesex, UK), followed by air drying for 1 week. Then, two batches of air-dried, 13 C-labelled GO were placed in a vial with water (15 ml), followed by addition of 15 N-labelled hydrazine monohydrate (98 atom% 15 N, Sigma-Aldrich; 1 μl for 3 mg of GO). The mixture was stirred at 80 °C for 1 day. After cooling to room temperature, the mixture was filtered using the Anodisc membrane filter, followed by air drying for 1 day, and finally dried under vacuum for 1 day. One batch of the sample (roughly 2 mg) was used to acquire the data as in Figures 1b , 2 . The second batch (10 mg), which had a lower degree of reduction, was used to acquire the data as in Figure 3 and Supplementary Figure S3 . Heat treatment of graphene oxide in water without hydrazine An aqueous suspension of unlabelled graphene oxide (3 mg of GO per 1 ml of purified water) was prepared by sonication of GO, prepared via the modified Hummers method and derived from natural graphite (SP-1, Bay Carbon) as described previously. This suspension was stirred at 80 °C for 12 h without hydrazine. The suspension was stable and the colour of the suspension was unchanged by the treatment. A paper-like material was prepared by filtration of the resulting suspension as previously reported [35] , [36] , and this material was used for XPS measurements. SSNMR measurements SSNMR experiments were conducted at 9.4 T using a Varian InfinityPlus 400 NMR spectrometer and a home-built 2.5-mm triple-resonance MAS probe at a 1 H NMR frequency of 400.214 MHz. All 13 C chemical shifts were referenced to tetramethylsilane using adamantane as an external reference. The 15 N chemical shifts were referenced to liquid 15 NH 3 at 0 p.p.m. using the indirect referencing of a 13 C signal for adamantane [40] , [41] . In all the experiments, the external air temperature was set to −10 °C using a Varian VT controller, and the MAS spinning speed was 20,000±10 Hz. For the measurement shown in Figure 1b , a 13 C single-pulse echo sequence was used with a π/2 pulse of 2.5-μs width and no 1 H decoupling. We confirmed that removing 1 H decoupling did not alter the resolution. A separate 13 C– 1 H REDOR experiment for the RGO sample confirmed that the peaks at 120 and 150 p.p.m. in Figure 1b could likely be associated with non-protonated carbons. Thus, fast spinning at 20 kHz sufficiently removed line broadening due to 1 H– 13 C dipolar couplings. For Figure 2a,b , a total of 5,400 scans were collected with recycle delays of 5 s and 15 N and 13 C π-pulse widths of 15 and 10 μs, respectively. A 13 C– 15 N REDOR pulse sequence ( Fig. 2d ) was used with a total of 32 rotor periods (1.6 ms) for dipolar dephasing. 1 H decoupling during the REDOR period was 55 kHz; we confirmed that there was little change in the spectra without 1 H decoupling. No 1 H decoupling was applied during the acquisition period. The spinning speed of 20,000±10 Hz was used to remove relatively strong 13 C– 13 C dipolar couplings. The π-pulse widths were 10 and 15 μs for 13 C and 15 N, respectively. In these REDOR experiments, the 13 C nuclei in the vicinity of 15 N nuclei lose their signals in the 13 C MAS spectrum with 13 C– 15 N dipolar dephasing. In a control REDOR experiment for uniformly 13 C- and 15 N-labelled L -alanine [24] , a signal for 13 C α that is directly bonded to 15 NH 3 + decreased by 78%, compared with the control spectrum without 13 C– 15 N dipolar dephasing. In the same study, signals for –CO 2 − and –CH 3 , which are two bonds away from 15 N, decreased by only 6 and 8%, respectively. The integrated intensity of the difference spectrum in Figure 2c is about 7.5±0.5% with respect to that of Figure 2a . Although the signal intensities in the experiment are modulated by 13 C– 13 C J-coupling and 13 C transverse spin relaxation, the result indicates that a considerable fraction of 13 C atoms observed here are likely to be bonded to 15 N species. Gaussian line broadening of 200 Hz was applied. For Figure 3a,b , a pulse sequence in Figure 3c was used. First, 15 N spin polarization was prepared by ramped CP [42] . Because of the limited population of the target 15 N species and a broad line width, the signal-to-noise ratio in the direct-detected 15 N CPMAS spectra was low even with 15 N enrichment. Thus, we used 1 H detected 15 N– 1 H double CP for the adjustment of the Hartmann–Hahn condition [43] , [44] . The 1 H polarization was excited by a 1 H π/2 pulse of 3.5-μs width. During a contact period of 0.35 ms for polarization transfer by CP, the 15 N radio-frequency (RF) field amplitude was linearly swept from 21 to 36 kHz, while the 1 H RF amplitude was kept constant at 48 kHz. 15 N and 13 C π-pulse widths in the REDOR sequence were 15 μs. The signals of 21,504 scans were accumulated with recycle delays of 3 s. Gaussian line broadening of 400 Hz was applied. The total experimental time was ~19 h for each sample. XPS measurements An aqueous suspension of graphene oxide was prepared by exfoliation of GO. The aqueous suspension (3.1 mg ml −1 ) was diluted with ethanol for facile spin casting onto glass substrates (Corning 1737). Graphene oxide thin films were prepared by spin casting the solution on a glass substrate cleaned by ultraviolet oxygen radiation. The films were subsequently reduced by a 1-h exposure to hydrazine vapour generated at 100 °C in a sealed container. One subset of the hydrazine vapour-treated samples was set aside for testing after the hydrazine vapour treatment. The remaining vapour-treated samples were reduced with thermal annealing at 750 °C in a CVD chamber under H 2 flow (100 sccm) for 5 min. Paper-like materials of reduced graphene oxide were prepared by simple filtration as previously reported [35] , [36] . Thermal annealing of the paper sample was done under Ar flow for 12 h at 500 °C. After the reduction process, surface chemical analysis of each reduced graphene oxide sample was performed by using XPS (Sigma Probe, Thermo VG Scientific). DFT calculations on the pyrazole formation For DFT calculations, we used the projector-augmented wave potentials [45] with a plane-wave basis set and the Perdew–Burke–Ernzernhof [46] exchange-correlation functional as implanted in the Vienna Ab-Initio Simulation Package [38] . A kinetic energy cutoff of 400 eV and Gaussian smearing of 0.05 eV was used. A (6×6) zigzag graphene nanoribbon supercell with vacuum separation of 10 Å and a (8×1×1) k -points sampling were used in calculations. All atomic forces were minimized at <0.025 eV Å −1 , and the in-plane stresses were fully relaxed. How to cite this article: Park, S. et al . Chemical structures of hydrazine-treated graphene oxide and generation of aromatic nitrogen doping. Nat. Commun. 3:638 doi: 10.1038/ncomms1643 (2012).